STAT3 restrains RANK- and TLR4-mediated signalling by suppressing expression of the E2 ubiquitin-conjugating enzyme Ubc13 The transcriptional regulator STAT3 curbs pro-inflammatory cytokine production mediated by NF-κB signalling in innate immune cells, yet the mechanism by which this occurs has been unclear. Here we identify STAT3 as a pivotal negative regulator of Ubc13, an E2 ubiquitin-conjugating enzyme that facilitates TRAF6 K63-linked ubiquitination and NF-κB activation. Ubc13 accumulates intracellularly in the absence of STAT3. Depletion of Ubc13 in Stat3 -deficient macrophages subdues excessive RANKL- or LPS-dependent gene expression, indicating that Ubc13 overexpression mediates enhanced transcriptional responses in the absence of STAT3. In RANKL-activated macrophages, STAT3 is stimulated by autocrine IL-6 and inhibits accrual of Ets-1, Set1 methyltransferase and trimethylation of histone H3 lysine 4 (H3K4me3) at the Ube2n (Ubc13) promoter. These results delineate a mechanism by which STAT3 operates as a transcriptional repressor on Ube2n , thus modulating NF-κB activity by regulation of Ubc13 abundance. Our data suggest that this pathway plays important roles in bone homeostasis and restraint of inflammation. Signal transducer and activator of transcription 3 (STAT3) is a cytokine-responsive transcription factor involved in important immune functions including both pro- and anti-inflammatory mechanisms [1] . A major unresolved question centres on how STAT3 restrains pro-inflammatory cytokine production from innate immune cells such as macrophages or dendritic cells (DCs) on Toll-like receptor (TLR) stimulation [2] , [3] . Conditional Stat3 deletion in murine myeloid or DC lineages, as well as pan-hematopoietic deletion, leads to intestinal inflammation resembling human inflammatory bowel disease [2] , [3] , [4] , underscoring the vital nature of the STAT3-mediated anti-inflammatory response. This response may be conserved, as humans with heterozygous inactivating STAT3 mutations in autosomal dominant hyper-immunoglobulin E syndrome (AD-HIES) present with immunodeficiency accompanied by disordered inflammation and elevated pro-inflammatory cytokines, a phenotype recapitulated in a mouse model of AD-HIES [5] , [6] , [7] . Strikingly, STAT3 deficiency in humans and mice also associates with bone abnormalities and elevated osteoclast amounts [5] , [8] , [9] suggesting effects on the receptor activator of nuclear factor κB (NF-κB; RANK) signalling pathway. By contrast, chronic STAT3 activation in tumour microenvironments induces immune suppression [10] , [11] . The underlying basis for the immunosuppressive and anti-inflammatory functions of STAT3 has been poorly understood. NF-κB signal transduction is necessary for TLR-triggered production of pro-inflammatory cytokines from myeloid cells and DCs. Like STAT3, NF-κB has numerous roles in immunity and development, and is frequently co-opted to regulate tumorigenesis and tumour-promoting inflammation [12] . NF-κB is activated by signalling cascades involving post-translational modifications including ubiquitination. Tumour necrosis factor (TNF) receptor-associated factor 6 (TRAF6) is a critical E3 ligase that mediates NF-κB signal transduction from TLRs as well as members of the TNF receptor superfamily such as RANK [13] . TRAF6 is activated on interaction with the ubiquitin-conjugating E2 enzyme Ubc13, which stimulates formation of the signal-promoting lysine 63 (K63)-linked polyubiquitination modification [14] . Ubc13 has been implicated in multiple cellular processes including inflammation [15] , although little is known about mechanisms that control its expression. The multifunctional cytokine IL-6 links the NF-κB and STAT3 signalling cascades in inflammatory and immune responses [16] . IL-6 production is triggered by NF-κB on TLR activation, a response that is often accompanied by concomitant generation of pro-inflammatory cytokines such as IL-1 and TNFα. IL-6 interacts with its cell surface gp130-containing receptor to elicit intracellular STAT3 and STAT1 signal transduction. Similar to STAT3, IL-6 has both pro- and anti-inflammatory roles [1] . For example, in cancer, IL-6 contributes to tumour-promoting inflammation, while endogenous IL-6 restrains osteoclastogenesis as well as the level of pro-inflammatory cytokines elicited during local or systemic acute inflammation [16] , [17] , [18] . Here we identify a new link between the STAT3 and NF-κB signalling pathways that may explain the anti-inflammatory function of STAT3. We found that IL-6-activated STAT3 functions as a transcriptional repressor for Ube2n , the gene encoding Ubc13. Thus, STAT3 inhibits accumulation of Ubc13 and thereby restrains NF-κB-mediated signalling responses. STAT3 suppresses RANK signalling and Ubc13 expression Previous studies indicated that hematopoietic Stat3 -deficient mice and individuals with AD-HIES due to STAT3 mutation develop osteoporotic phenotypes [9] , [19] . We found that tartrate-resistant acid phosphatase-positive (TRAP + ) osteoclasts are present in greater abundance in femurs from hematopoietic Stat3 -deficient mice compared with Stat3 -sufficient animals. Moreover, Stat3 -deficient bone marrow-derived macrophages showed an increased propensity to form osteoclasts in RANK-ligand (RANKL) cultures ( Fig. 1a,b ). These results suggest that Stat3 deficiency enables elevated responses to RANKL. Stat3 deficiency in hematopoietic cells also renders heightened TLR4 signalling [2] . TLR4 and RANK responses rely on NF-κB activation through the adaptor protein TRAF6 (ref. 13 ), suggesting a common mechanism of STAT3 function that converges on TRAF6. We therefore examined RANK signal transduction to TRAF6 in bone marrow-derived macrophages. Our results show enhanced total and K63-linked ubiquitination of TRAF6 in Stat3 -deficient macrophages on RANKL stimulation, relative to Stat3 -sufficient controls ( Fig. 1c,d ). TRAF6 induces activation of NF-κB as well as the mitogen-activated protein kinase (MAPK) cascade downstream of RANK or TLR4 (ref. 20 ). We detected increased RANKL-stimulated NF-κB DNA-binding activity in Stat3 -deficient macrophages, without effects on RANK or macrophage marker protein expression ( Fig. 1e ; Supplementary Fig.1 ). Moreover, c-Jun N-terminal kinase (JNK) and p38 activation by RANKL was increased in the absence of STAT3 ( Fig. 1f ). These results suggest that STAT3 restrains the amplitude and duration of signal transduction pathways activated by RANKL by modulating K63-linked ubiquitination of TRAF6. 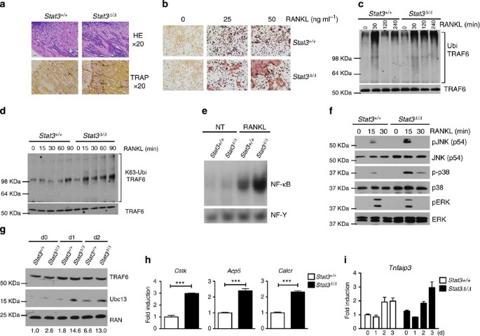Figure 1: STAT3 suppresses osteoclastogenesis and RANK signal transduction. (a) Femoral sections fromStat3-deficient (Stat3Δ/Δ) and -sufficient (Stat3+/+) mice, 8 weeks. (Upper) Hematoxylin and eosin (HE); (lower) TRAP staining (arrows). Scale bar, 100 μM. (b–i) Bone marrow cells fromStat3+/+andStat3Δ/Δmice were cultured in M-CSF-containing medium for 4 days to generate bone marrow-derived macrophages. (b) Cells (2 × 105) were cultured in M-CSF and RANKL (0, 25 or 50 ng ml−1) for an additional 4 days. Osteoclasts detected by TRAP staining (pink). Scale bar, 100 μM. (c–f) Macrophages were starved of exogenous growth factor overnight and stimulated with RANKL (100 ng ml−1) or left untreated, as indicated. (c,d) TRAF6 ubiquitination was evaluated −/+ RANKL stimulation by immunoprecipitation and immunoblotting for total ubiquitin (c) or K63-specific linkage (d). Lower panels: total TRAF6. (e) NF-κB DNA-binding activity was measured −/+ RANKL stimulation (15 min) by electrophoretic mobility shift assay (EMSA). Loading control: NF-Y EMSA. (f) MAPK activation was measured −/+ RANKL stimulation by immunoblotting whole-cell lysates with antibodies specific for phosphorylated protein (pJNK, p-p38 or pERK). Total protein amounts served as loading controls (JNK, p38 or ERK). (g) Macrophages were cultured in M-CSF and RANKL (50 ng ml−1). TRAF6 and Ubc13 amounts were determined by immunoblotting. Loading control: RAN. The relative level of Ubc13 is expressed as a ratio of Ubc13:RAN at each time point (indicated below bottom panel); amounts inStat3+/+cells on day 0=1.0 fold (arbitrary unit). (h) Macrophages were cultured in M-CSF and RANKL (50 ng ml−1) for 3 days. Expression of osteoclast genesCstk,Acp5andCalcrwas determined by qPCR. Relative mRNA amounts for each gene expressed as fold induction versus expression inStat3-sufficient cells. (i) A20 (Tnfaip3) expression was determined after culturing macrophages in M-CSF and RANKL (50 ng ml−1) for 0, 1, 2 or 3 days, using qPCR. (a) Results representn=5 per genotype. (b–g) Results represent three independent experiments. (h,i) Data represent mean values of three independent experiments. Error bars indicate s.e.m. (h)t-test used; ***P<0.001 for indicated comparisons. (i) Two-way ANOVA with Bonferroni multiple comparison used; not significant. Figure 1: STAT3 suppresses osteoclastogenesis and RANK signal transduction. ( a ) Femoral sections from Stat3 -deficient ( Stat3 Δ/Δ ) and -sufficient ( Stat3 +/+ ) mice, 8 weeks. (Upper) Hematoxylin and eosin (HE); (lower) TRAP staining (arrows). Scale bar, 100 μM. ( b – i ) Bone marrow cells from Stat3 +/+ and Stat3 Δ/Δ mice were cultured in M-CSF-containing medium for 4 days to generate bone marrow-derived macrophages. ( b ) Cells (2 × 10 5 ) were cultured in M-CSF and RANKL (0, 25 or 50 ng ml −1 ) for an additional 4 days. Osteoclasts detected by TRAP staining (pink). Scale bar, 100 μM. ( c – f ) Macrophages were starved of exogenous growth factor overnight and stimulated with RANKL (100 ng ml −1 ) or left untreated, as indicated. ( c , d ) TRAF6 ubiquitination was evaluated −/+ RANKL stimulation by immunoprecipitation and immunoblotting for total ubiquitin ( c ) or K63-specific linkage ( d ). Lower panels: total TRAF6. ( e ) NF-κB DNA-binding activity was measured −/+ RANKL stimulation (15 min) by electrophoretic mobility shift assay (EMSA). Loading control: NF-Y EMSA. ( f ) MAPK activation was measured −/+ RANKL stimulation by immunoblotting whole-cell lysates with antibodies specific for phosphorylated protein (pJNK, p-p38 or pERK). Total protein amounts served as loading controls (JNK, p38 or ERK). ( g ) Macrophages were cultured in M-CSF and RANKL (50 ng ml −1 ). TRAF6 and Ubc13 amounts were determined by immunoblotting. Loading control: RAN. The relative level of Ubc13 is expressed as a ratio of Ubc13:RAN at each time point (indicated below bottom panel); amounts in Stat3 +/+ cells on day 0=1.0 fold (arbitrary unit). ( h ) Macrophages were cultured in M-CSF and RANKL (50 ng ml −1 ) for 3 days. Expression of osteoclast genes Cstk , Acp5 and Calcr was determined by qPCR. Relative mRNA amounts for each gene expressed as fold induction versus expression in Stat3 -sufficient cells. ( i ) A20 ( Tnfaip3 ) expression was determined after culturing macrophages in M-CSF and RANKL (50 ng ml −1 ) for 0, 1, 2 or 3 days, using qPCR. ( a ) Results represent n =5 per genotype. ( b – g ) Results represent three independent experiments. ( h , i ) Data represent mean values of three independent experiments. Error bars indicate s.e.m. ( h ) t -test used; *** P <0.001 for indicated comparisons. ( i ) Two-way ANOVA with Bonferroni multiple comparison used; not significant. Full size image Total TRAF6 protein amounts did not vary on RANKL treatment ( Fig. 1c,d ), suggesting that an additional factor mediates enhanced RANKL signalling in Stat3 -deficient cells. We found that Ubc13 expression was higher in Stat3 -deficient macrophages under basal conditions and was substantially increased in response to RANKL relative to Stat3 -sufficient controls ( Fig. 1g ), correlating with elevated RANKL-dependent signal transduction and osteoclast gene expression ( Fig. 1c–f,h ). To examine mechanisms that lead to Ubc13 accumulation, we investigated A20, a deubiquitinase that triggers proteasome-dependent degradation of Ubc13 and negatively regulates TRAF6-mediated NF-κB and MAPK activation [21] . We found that A20 was induced by RANKL similarly in the absence or presence of STAT3 ( Fig. 1i ), indicating that A20 is not involved in the STAT3-dependent mechanism that restrains Ubc13 expression and RANKL signalling in macrophages. Together, our results suggest that Ubc13 accumulation in Stat3 -deficient cells is an important response, regulated independently of A20, which results in augmented RANKL and inflammatory signal transduction. RANK and TLR4 signalling is enhanced by Ubc13 upregulation To examine involvement of Ubc13, we investigated the effects of manipulating its expression in Stat3 -deficient cells. We generated mice that contained a tamoxifen-inducible cre transgene and floxed alleles of Ube2n (Ubc13) and Stat3 . Using bone marrow cells from these animals, we deleted Ube2n and Stat3 ex vivo in bone marrow-derived macrophages and investigated signalling responses to RANKL and lipopolysaccharide (LPS). We found that concomitant Ube2n and Stat3 deletion repressed expression of RANKL- or LPS-induced genes to levels at or below those found in Stat3 -sufficent cells ( Fig. 2a,b ), indicating a central non-redundant role for Ubc13 in rendering elevated transcriptional responses in the absence of STAT3. Importantly, short hairpin RNA (shRNA)-mediated knockdown of Ubc13 in Stat3 -deficient macrophages, to amounts found in Stat3 -sufficient cells, decreased RANKL- or LPS-dependent gene expression to levels observed in the presence of STAT3 ( Supplementary Fig. 2a–c ). Since Ubc13 expression in knockdown conditions approximated levels present in Stat3 -sufficient cells, the results suggest accumulated Ubc13 as a major factor in the excessive RANKL- or LPS-mediated transcriptional response elicited in the absence of STAT3. By contrast, enforced Ubc13 overexpression in Stat3 -sufficient macrophages rendered substantially elevated osteoclast-specific mRNA expression in response to RANKL ( Supplementary Fig. 2d,e ), confirming that increases in Ubc13 amounts result in enhanced gene expression. 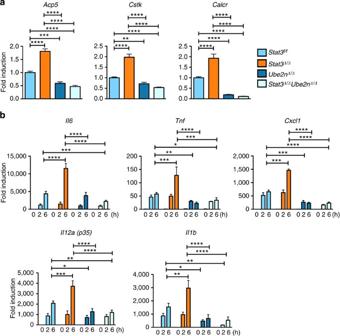Figure 2: Ubc13 mediates enhanced RANKL- and LPS-responsive gene expression induced byStat3-deficiency. Bone marrow cells fromStat3f/f, Cre-ERStat3f/f, Cre-ERUbe2nf/for Cre-ERStat3f/fUbe2nf/fmice were cultured in M-CSF-containing media plus 4-hydroxytamoxifen for 4 days to generateStat3-sufficient (Stat3f/f),Stat3-deficient (Stat3Δ/Δ),Ube2n-deficient (Ube2nΔ/Δ) orStat3-deficient,Ube2n-deficient (Stat3Δ/ΔUbe2nΔ/Δ) macrophages, respectively. Cells were cultured in M-CSF- and RANKL-containing medium for 3 days (a) or stimulated with LPS (b), as indicated. Gene expression was analysed by qPCR. Results represent mean values of three independent experiments. Error bars indicate s.e.m. Two-way ANOVA with Bonferroni multiple comparison used. *P<0.05; **P<0.01; ***P<0.001; ****P<0.0001 for indicated comparisons. Figure 2: Ubc13 mediates enhanced RANKL- and LPS-responsive gene expression induced by Stat3 -deficiency. Bone marrow cells from Stat3 f/f , Cre-ER Stat3 f/f , Cre-ER Ube2n f/f or Cre-ER Stat3 f/f Ube2n f/f mice were cultured in M-CSF-containing media plus 4-hydroxytamoxifen for 4 days to generate Stat3 -sufficient ( Stat3 f/f ), Stat3 -deficient ( Stat3 Δ/Δ ), Ube2n- deficient ( Ube2n Δ/Δ ) or Stat3- deficient, Ube2n -deficient ( Stat3 Δ/Δ Ube2n Δ/Δ ) macrophages, respectively. Cells were cultured in M-CSF- and RANKL-containing medium for 3 days ( a ) or stimulated with LPS ( b ), as indicated. Gene expression was analysed by qPCR. Results represent mean values of three independent experiments. Error bars indicate s.e.m. Two-way ANOVA with Bonferroni multiple comparison used. * P <0.05; ** P <0.01; *** P <0.001; **** P <0.0001 for indicated comparisons. Full size image STAT3 also stimulates the inhibitor suppressor of cytokine signalling 3 (SOCS3), which facilitates interaction of signalling proteins with the ubiquitin-mediated degradation pathway [1] , [22] . This raised the possibility that SOCS3 contributes to repression of Ubc13. We ruled out SOCS3 involvement by observing that enforced SOCS3 expression in Stat3 -deficient cells did not affect Ubc13 protein abundance or LPS-dependent gene expression ( Supplementary Fig. 3a,b ). In comparison, STAT3 overexpression in Stat3 -deficient cells reduced LPS-dependent gene expression and Ubc13 protein amounts ( Supplementary Fig. 3c,d ). Therefore, our data implicate Ubc13 as a key factor in the pathway by which STAT3 dampens RANKL- and LPS-mediated gene expression. Autocrine IL-6-STAT3 signalling represses Ubc13 expression We next addressed the nature of the signal that induces STAT3 activity and the mechanism by which STAT3 controls Ubc13 expression. We noted that IL-6 inhibits osteoclastogenesis [17] . This suggested that an IL-6-STAT3 autocrine loop might suppress Ubc13 amounts and RANKL-mediated signalling. We found that RANKL induced Il6 mRNA in macrophages ( Fig. 3a ). To test whether autocrine IL-6 regulated RANKL signalling, we used IL-6 antibody blockade or Il6 −/− cells. We found IL-6 neutralization by antibody blockade enhanced RANKL-responsive osteoclast gene expression and Ubc13 protein amounts in bone marrow-derived macrophages ( Fig. 3b,c ). Moreover, Il6 −/− macrophages showed elevated Ubc13 protein amounts, NF-κB activity and osteoclast gene expression following RANKL treatment ( Fig. 3d–f ). By contrast, stimulation with recombinant IL-6 suppressed Ubc13 amounts in Stat3 -sufficient but not Stat3 -deficient cells ( Fig. 3g ; Supplementary Fig. 3d ). Collectively, our results indicate that IL-6 triggers STAT3-dependent repression of Ubc13 expression, inhibiting RANKL- and LPS-induced signalling. 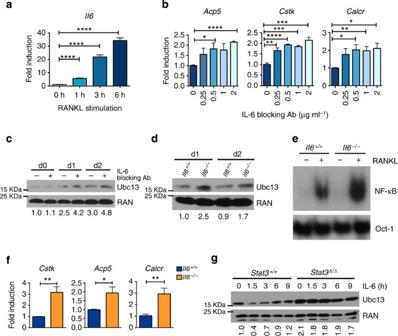Figure 3: Autocrine IL-6 is required to repress Ubc13 expression. (a)Il6mRNA expression was measured in bone marrow-derived macrophages by qPCR following RANKL (50 ng ml−1) stimulation, as indicated. (b,c) Osteoclast gene expression (b) and Ubc13 amounts (c) were determined in bone marrow-derived macrophages following culture in M-CSF- and RANKL-containing medium without (−) or with (+) IL-6-blocking antibody by qPCR or immunoblotting, respectively. (d–f) Ubc13 amounts, NF-κB DNA-binding activity and osteoclast gene expression were determined inIl6+/+andIl6−/−bone marrow-derived macrophages following culture in M-CSF- and RANKL-containing medium for 1 or 2 days (d), 1 day (e) or 3 days (f) by immunoblotting, electrophoretic mobility shift assay or qPCR, respectively. (g) Ubc13 expression was evaluated in bone marrow-derived macrophages fromStat3-sufficient (Stat3+/+) or hematopoieticStat3-deficient (Stat3Δ/Δ) mice by immunoblotting following IL-6 stimulation, as indicated. (c,d,g) Relative Ubc13 expression versus untreated (c), IL-6- (d) or STAT3-sufficient control (g) was calculated as indicated inFig. 1gand displayed below bottom panels. (a,b,f) Results represent mean values of three independent experiments. Error bars indicate s.e.m. (a,b) Two-way ANOVA with Bonferroni multiple comparison used; (f)t-test used. *P<0.05; **P<0.01; ***P<0.001; ****P<0.0001 for indicated comparisons. (c,d,e,g) Results represent three independent experiments. Figure 3: Autocrine IL-6 is required to repress Ubc13 expression. ( a ) Il6 mRNA expression was measured in bone marrow-derived macrophages by qPCR following RANKL (50 ng ml −1 ) stimulation, as indicated. ( b , c ) Osteoclast gene expression ( b ) and Ubc13 amounts ( c ) were determined in bone marrow-derived macrophages following culture in M-CSF- and RANKL-containing medium without (−) or with (+) IL-6-blocking antibody by qPCR or immunoblotting, respectively. ( d – f ) Ubc13 amounts, NF-κB DNA-binding activity and osteoclast gene expression were determined in Il6 +/+ and Il6 −/− bone marrow-derived macrophages following culture in M-CSF- and RANKL-containing medium for 1 or 2 days ( d ), 1 day ( e ) or 3 days ( f ) by immunoblotting, electrophoretic mobility shift assay or qPCR, respectively. ( g ) Ubc13 expression was evaluated in bone marrow-derived macrophages from Stat3 -sufficient ( Stat3 +/+ ) or hematopoietic Stat3 -deficient ( Stat3 Δ/Δ ) mice by immunoblotting following IL-6 stimulation, as indicated. ( c , d , g ) Relative Ubc13 expression versus untreated ( c ), IL-6- ( d ) or STAT3-sufficient control ( g ) was calculated as indicated in Fig. 1g and displayed below bottom panels. ( a , b , f ) Results represent mean values of three independent experiments. Error bars indicate s.e.m. ( a , b ) Two-way ANOVA with Bonferroni multiple comparison used; ( f ) t -test used. * P <0.05; ** P <0.01; *** P <0.001; **** P <0.0001 for indicated comparisons. ( c , d , e , g ) Results represent three independent experiments. Full size image STAT3 utilizes a transcriptional mechanism to restrain Ube2n Previous studies indicated that the anti-inflammatory function of STAT3 relies on transcription, eliciting a response that dampens NF-κB signalling [23] . We found that direct stimulation of cells with recombinant IL-6 repressed Ube2n (Ubc13) mRNA amounts in macrophages, in addition to its inhibitory effects on Ubc13 protein ( Figs 3g and 4a ), suggesting potential to suppress Ube2n transcription. Moreover, IL-10, the classic anti-inflammatory cytokine utilizing STAT3, similarly dampens Ube2n mRNA amounts ( Supplementary Fig. 4a ). To examine whether STAT3 inhibits Ube2n transcription, we inspected the Ube2n promoter sequence. We identified a conserved STATx consensus site within 100 bp (base pair) of the predicted Ube2n transcriptional start site (TSS; Supplementary Fig. 4b ). Using reporter gene assays to test the function of this conserved STATx element, we found that STAT3 inhibited activity of the Ube2n promoter, while mutation of the STATx binding site abolished STAT3-mediated repression ( Fig. 4b ). These data suggest that STAT3 mediates transcriptional repression of Ube2n via the STATx site located near the TSS. 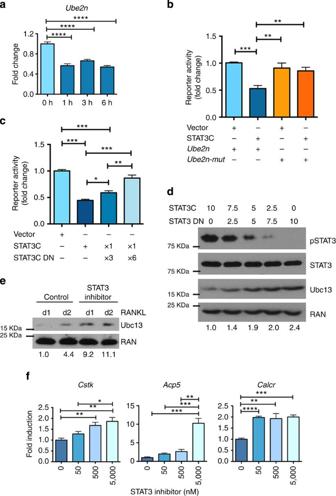Figure 4: STAT3 transcriptional activity is required to repressUbe2nexpression. (a)Ube2nmRNA was measured in bone marrow-derived macrophages fromStat3-sufficient mice following treatment with IL-6 as indicated, using qPCR. (b,c)Ube2npromoter activity was measured by reporter assays in HEK293T cells transfected with pGL3-Ube2n(Ube2n), pGL3-Ube2n-mut (Ube2n-mut; containing a mutated STATx site), pMX vector (vector), pMX-STAT3C (STAT3C), pMX-STAT3 DN (STAT3 DN) and pTK-Renilla, as indicated. pMX-STAT3 DN and pMX-STAT3C were included in some samples in a 3:1 or 6:1 ratio, as shown. (d)Stat3−/−MEFs were transfected with pMX-STAT3C, pMX-STAT3 DN or both, at the ratios indicated. The expression level of pSTAT3, total STAT3 and Ubc13 was detected by immunoblotting. RAN served as loading control. (e,f) Bone marrow-derived macrophages fromStat3-sufficient mice were cultured in M-CSF- and RANKL-containing medium in the absence or presence of the STAT3 inhibitor PM-73G, as indicated. Ubc13 amounts were detected by immunoblotting (e); osteoclast gene expression was measured by qPCR (f). (d,e) Relative Ubc13 expression versus STAT3C transfection alone (d) or untreated cells on 1 day (e) was calculated as indicated inFig. 1gand displayed below bottom panels. (a,b,c,f) Data represent mean values of three independent experiments. Error bars indicate s.e.m. Two-way ANOVA with Bonferroni multiple comparison used. *P<0.05; **P<0.01; ***P<0.001; ****P<0.0001 for the indicated comparisons. (d,e) Results represent three independent experiments. Figure 4: STAT3 transcriptional activity is required to repress Ube2n expression. ( a ) Ube2n mRNA was measured in bone marrow-derived macrophages from Stat3 -sufficient mice following treatment with IL-6 as indicated, using qPCR. ( b , c ) Ube2n promoter activity was measured by reporter assays in HEK293T cells transfected with pGL3- Ube2n ( Ube2n ), pGL3- Ube2n -mut ( Ube2n -mut; containing a mutated STATx site), pMX vector (vector), pMX-STAT3C (STAT3C), pMX-STAT3 DN (STAT3 DN) and pTK-Renilla, as indicated. pMX-STAT3 DN and pMX-STAT3C were included in some samples in a 3:1 or 6:1 ratio, as shown. ( d ) Stat3 −/− MEFs were transfected with pMX-STAT3C, pMX-STAT3 DN or both, at the ratios indicated. The expression level of pSTAT3, total STAT3 and Ubc13 was detected by immunoblotting. RAN served as loading control. ( e , f ) Bone marrow-derived macrophages from Stat3 -sufficient mice were cultured in M-CSF- and RANKL-containing medium in the absence or presence of the STAT3 inhibitor PM-73G, as indicated. Ubc13 amounts were detected by immunoblotting ( e ); osteoclast gene expression was measured by qPCR ( f ). ( d , e ) Relative Ubc13 expression versus STAT3C transfection alone ( d ) or untreated cells on 1 day ( e ) was calculated as indicated in Fig. 1g and displayed below bottom panels. ( a , b , c , f ) Data represent mean values of three independent experiments. Error bars indicate s.e.m. Two-way ANOVA with Bonferroni multiple comparison used. * P <0.05; ** P <0.01; *** P <0.001; **** P <0.0001 for the indicated comparisons. ( d , e ) Results represent three independent experiments. Full size image To further evaluate the mechanism by which STAT3 suppresses Ube2n transcription, we used STAT3 isoforms with mutations in regions that mediate transcriptional function. Overexpression of a STAT3 mutant with defective DNA-binding activity (STAT3 DN) attenuated the repressive effects of STAT3 signalling on Ube2n reporter activity as well as Ubc13 protein amounts ( Fig. 4c,d ). In addition, we found that the carboxy-terminal transactivation domain (TAD) was required for the inhibitory effect of STAT3 on Ube2n promoter activity ( Supplementary Fig. 5 ). Blockade of STAT3 SH2 domain function with PM-73G, a small-molecule phosphopeptide-based STAT3 inhibitor [24] , led to suppressed STAT3 tyrosine phosphorylation, accumulation of Ubc13 and enhanced RANKL-dependent gene expression ( Fig. 4e,f ; Supplementary Fig. 6a ). Moreover, STAT3 V637M, an SH2 domain mutant associated with AD-HIES [6] , mediated enhanced LPS-dependent inflammatory gene expression compared with wild-type STAT3 ( Supplementary Fig. 6b ). Taken together, our data suggest that STAT3 acts as a transcriptional repressor via its classic pathway (that is, SH2-dependent dimerization, DNA binding and trans -mediated events) to inhibit Ube2n /Ubc13 expression and modulate RANKL and inflammatory signalling responses. Ube2n repression coincides with Ets-1 and Set1 displacement To evaluate whether STAT3 acts directly as a transcriptional repressor on the Ube2n promoter, we examined whether STAT3 interacts with the promoter STATx site in vivo . By performing STAT3 chromatin immunoprecipitations (ChIPs) and quantitative PCR (qPCR), we found that IL-6 induced STAT3 binding to the Ube2n promoter in proximity to the conserved STATx site ( Fig. 5a,b ). Similarly, IL-10 stimulation resulted in STAT3 interaction with the Ube2n promoter within the region of the STATx element ( Fig. 5a,c ). These results indicate cytokine-induced STAT3 accumulation at the Ube2n promoter, which correlates with reduced mRNA expression, suggesting a direct mechanism of Ube2n transcriptional repression. 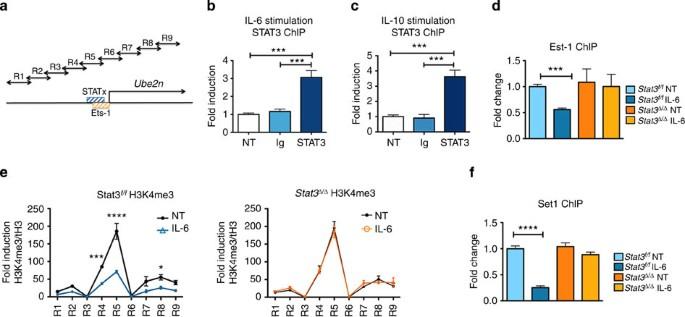Figure 5: STAT3 repressesUbe2ntranscription by regulating Ets-1 association and H3K4me3 abundance at the proximal promoter. (a) Schematic diagram showing the approximate location of the putative STATx (blue) and Ets-1 consensus sites (orange) and primers used for H3K4me3 ChIPs (arrows, sequences are listed inSupplementary Table I). (b,c) STAT3 association with theUbe2npromoter was measured by ChIPs fromStat3-sufficient bone marrow-derived macrophages in the absence (NT) or presence of IL-6 (b) or IL-10 (c) stimulation for 1 h, as indicated. IgG ChIPs were performed as control. (d–f) Bone marrow cells fromStat3f/for Cre-ERStat3f/fmice were cultured in M-CSF-containing media and 4-hydroxytamoxifen for 5 days to generateStat3-sufficient (Stat3f/f) orStat3-deficient (Stat3Δ/Δ) macrophages, respectively. Association of Ets-1 (d), H3K4me3 (e) or Set1 (f) with theUbe2npromoter in the vicinity of the STAT3-binding site (d,f) or theUbe2nproximal promoter (±1 kb of TSS;e) was measured by ChIPs, with (IL-6) or without (NT) IL-6 stimulation for 1 h, as indicated. ChIP primers for R5 were used ford,f. (b–f) Data represent mean values of three independent experiments. Error bars indicate s.e.m. Two-way ANOVA with Bonferroni multiple comparison used. *P<0.05; ***P<0.001; ****P<0.0001 for the indicated comparisons. Figure 5: STAT3 represses Ube2n transcription by regulating Ets-1 association and H3K4me3 abundance at the proximal promoter. ( a ) Schematic diagram showing the approximate location of the putative STATx (blue) and Ets-1 consensus sites (orange) and primers used for H3K4me3 ChIPs (arrows, sequences are listed in Supplementary Table I ). ( b , c ) STAT3 association with the Ube2n promoter was measured by ChIPs from Stat3 -sufficient bone marrow-derived macrophages in the absence (NT) or presence of IL-6 ( b ) or IL-10 ( c ) stimulation for 1 h, as indicated. IgG ChIPs were performed as control. ( d – f ) Bone marrow cells from Stat3 f/f or Cre-ER Stat3 f/f mice were cultured in M-CSF-containing media and 4-hydroxytamoxifen for 5 days to generate Stat3 -sufficient ( Stat3 f/f ) or Stat3 -deficient ( Stat3 Δ/Δ ) macrophages, respectively. Association of Ets-1 ( d ), H3K4me3 ( e ) or Set1 ( f ) with the Ube2n promoter in the vicinity of the STAT3-binding site ( d , f ) or the Ube2n proximal promoter (±1 kb of TSS; e ) was measured by ChIPs, with (IL-6) or without (NT) IL-6 stimulation for 1 h, as indicated. ChIP primers for R5 were used for d , f . ( b – f ) Data represent mean values of three independent experiments. Error bars indicate s.e.m. Two-way ANOVA with Bonferroni multiple comparison used. * P <0.05; *** P <0.001; **** P <0.0001 for the indicated comparisons. Full size image We considered potential scenarios for STAT3-mediated transcriptional repression, including whether cytokine-inducible STAT3 binding might affect constitutive association of transcriptional regulators at the Ube2n promoter. Further inspection of the Ube2n promoter revealed an Ets consensus sequence that overlapped with the STATx site ( Fig. 5a ; Supplementary Fig. 4b ). Using ChIPs, we found that the transcription factor Ets-1 was localized to the Ube2n promoter in the absence of cytokine stimulation ( Fig. 5d ). Ets-1 binding was reduced on IL-6 stimulation in Stat3 -sufficient but not Stat3 -deficient cells ( Fig. 5d ), suggesting that STAT3 mediates the decrease in Ets-1 association at the Ube2n promoter in response to cytokine treatment. A recent study showed genome-wide Ets-1 binding in proximity to the chromatin modification H3K4me3, which is linked to transcriptional activation [25] . We analysed effects of IL-6-STAT3 signalling on H3K4me3 at the Ube2n promoter by measuring H3K4me3 abundance across a 2-kb region centred on the Ube2n TSS. We found that IL-6 reduced H3K4me3 amounts at the Ube2n TSS, relative to unstimulated cells ( Fig. 5a,e ). Furthermore, we found that IL-6-dependent H3K4me3 repression at the Ube2n TSS required STAT3, as indicated by the lack of suppression in Stat3 -deficient macrophages ( Fig. 5e ). Significantly, the IL-6-STAT3-dependent reduction in H3K4me3 occurred in the region that STAT3 and Ets-1 occupy ( Fig. 5a,b,d ). The H3K4me3 modification is deposited by Set domain-containing methyltransferases [26] . Accordingly, we assayed Set1 binding to the Ube2n promoter region by ChIPs. We found Set1 associated with the Ube2n promoter in the absence of IL-6 stimulation, while IL-6 signalling decreased Set1 accumulation in Stat3 -sufficient but not Stat3 -deficient cells ( Fig. 5f ), implying that STAT3 is involved in IL-6-dependent reduction in Set1. Collectively, our results suggest that STAT3 acts as a cytokine-inducible transcriptional repressor at the Ube2n promoter, leading to displacement of constitutively associated Ets-1, reduction in Set1 abundance and decreased amounts of the transcriptionally active H3K4me3 modification. Here we demonstrate that STAT3 represses Ubc13 expression by direct transcriptional inhibition, causing restraint of TRAF6 K63-linked ubiquitination, NF-κB signalling and RANKL- and LPS-responsive gene expression. To our knowledge, these results provide the first mechanistic description of how STAT3 operates as a transcriptional repressor. Furthermore, they reveal an important molecular pathway by which STAT3 exerts anti-inflammatory activity and suppresses osteoclastogenesis [1] . Our data may explain why hematopoietic Stat3 -deficient mice and humans with heterozygous STAT3 inactivating mutations and AD-HIES have increased inflammatory cytokine expression and skeletal abnormalities such as recurrent bone fractures [5] , [6] , [8] . By contrast, STAT3-mediated repression of Ubc13 may contribute to autocrine or paracrine effects of persistent IL-6-STAT3 signalling in disease, including cancer-promoting immune suppression [10] , [11] . Manipulating the STAT3-Ubc13 axis might be an approach to influence inflammatory responses for therapeutic benefit. An anti-inflammatory role for STAT3 has been observed for decades, without the molecular basis of this function understood. Previous studies showed that the anti-inflammatory activity is generated from a wide variety of STAT3-activating receptors, including natural as well as engineered receptors [27] , indicating a general signalling role for STAT3. Moreover, compelling evidence suggests that STAT3 acts as a transcription factor to regulate the anti-inflammatory response [23] . Accordingly, STAT3 inhibits NF-κB family members from stimulating transcription at specific gene promoters such as Il12p40 and Bcl3 (refs 28 , 29 ); however, these data do not fully explain the wide-ranging anti-inflammatory activity of STAT3. By identifying Ube2n as a STAT3-repressed gene, we reveal a mechanism that has a broad effect on Ubc13/TRAF6-mediated signalling to NF-κB, which may explain the molecular basis of the general STAT3 anti-inflammatory response. Our studies highlight an important role for autocrine IL-6-activated STAT3 in restraining RANKL- and LPS-induced gene expression. While this is consistent with the known function of IL-6 in suppressing in vitro osteoclastogenesis, IL-6 has complex effects on bone formation and resorption including promotion of RANKL production from osteoblasts and induction of myeloid progenitors that can serve as osteoclast precursors (for example, colony-forming unit granulocyte–macrophage). Furthermore, the Il6 -deficient strain we utilized for in vitro studies may contribute to the effects observed on RANKL signalling, and thus additional work is required to confirm results in vivo [5] , [8] , [9] , [17] , [30] . Moreover, IL-6 is frequently described as a pro- versus anti-inflammatory cytokine. This characterization appears to be context specific as IL-6 elicits both pro- and anti-inflammatory activities in vivo [16] , [17] , [18] . In fact, recent work underscores the importance of the IL-6 anti-inflammatory function in mediating macrophage alternative activation [31] . By contrast, IL-10 is the archetypal anti-inflammatory cytokine, activity that is attributed to exclusive activation of STAT3 through the IL-10 receptor [23] , [32] . Importantly, we found that IL-10 also recruits STAT3 to the Ube2n promoter and suppresses Ube2n mRNA, consistent with Ubc13 repression as a key component of STAT3 anti-inflammatory signalling. Our results, however, failed to support a major function of SOCS3 in curbing LPS-dependent gene responses. SOCS3 has been proposed to mediate the anti-inflammatory function of STAT3, yet Socs3 gene ablation in mice is protective against LPS-induced sepsis shock [33] . Moreover, mutation of the SOCS3-binding site in gp130, the signalling subunit of the IL-6 receptor, enhanced the anti-inflammatory activity of IL-6 (refs 27 , 33 ). Together, these data indicate that SOCS3 restrains anti-inflammatory signalling, consistent with its role as a general inhibitor of cytokine signal transduction, blocking downstream Janus kinase and STAT activity. Thus, the collective data are consistent with a potent anti-inflammatory response elicited by STAT3-dependent repression of Ubc13, which may be enhanced by SOCS3 removal. STATs were first identified as transcriptional activators, although it is increasingly clear that certain STATs also function to repress expression of specific genes [34] , [35] . Here, to our knowledge, we report the first detailed description of a mechanism by which STAT3 acts as a transcriptional repressor. Our data suggest that STAT3 operates via its classical signalling pathway, including SH2-domain-mediated dimerization and DNA binding to suppress Ube2n transcription. STAT3 association at the Ube2n promoter is accompanied by inhibition of constitutive Ets-1 binding, reduced amounts of the transcriptionally active chromatin mark H3K4me3 and Set1 association. This suggests at least two potential mechanisms for Ube2n inhibition: direct competition between STAT3 and Ets-1 for Ube2n promoter binding or indirect displacement of Ets-1 by an as yet unknown STAT3-recruited factor(s). Either scenario would be consistent with requirements for STAT3 SH2, DNA binding and TAD, and will require further investigation to resolve. Moreover, while our results suggest that Ets-1 mediates Ube2n transcriptional activation and, potentially, Set1 association along with H3K4me3 accumulation, these mechanisms of Ube2n regulation remain to be tested directly. Significantly, the co-localization of STATx- and Ets-1-binding sites at the Ube2n / UBE2N promoter is conserved between mice and humans, suggesting that murine and human STAT3 may function to repress Ube2n / UBE2N similarly. In accordance, AD-HIES patients contain mutations in STAT3 domains involved in transcriptional activity, show bone abnormalities consistent with enhanced osteoclastogenesis and exhibit features of deregulated inflammation [5] , [8] . Thus, while our data suggest that the RANKL-inhibiting and anti-inflammatory role for murine STAT3 is mediated by Ets-1 displacement on the Ube2n promoter, it is important to determine whether this mechanism operates on human UBE2N , if it occurs at other STAT3-repressed genes, and if it represents a genome-wide response to STAT3 signalling that coordinates other critical biological activities. IL-6 is widely recognized as an important cancer-promoting cytokine. This activity is attributed to its ability to stimulate proliferation of malignant epithelial cells and induce a pro-tumorigenic microenvironment by enhancing angiogenesis and expansion of myeloid-derived suppressor cells, tumour-associated macrophages and CD4 + IL-17-secreting cells [36] . Thus, therapeutic inhibition of the IL-6-STAT3 signalling axis, with both IL-6- and IL-6Rα-blocking antibodies, has become a major goal, particularly for cancers induced or promoted by chronic inflammation [36] . As a STAT3-repressed gene, Ube2n expression levels would be expected to increase in the presence of IL-6 or STAT3 inhibitors. Accordingly, we observed Ubc13 upregulation in bone marrow-derived macrophages treated with a peptide-based STAT3 inhibitor, as well as Ube2n- induction in lung myeloid cell infiltrates on delivery of IL-6-blocking antibodies in a mutant K-ras lung cancer model in vivo , a treatment that has a positive correlation with tumour suppression (unpublished work). These results suggest the potential for increases in Ubc13 in myeloid cells to be protective and elicit anti-tumour responses in the tumour environment. In addition, while our studies focused on myeloid responses, the fact that Ubc13 is restrained by STAT3 in murine embryonic fibroblasts (MEFs) suggests that the STAT3-Ubc13 pathway may operate in non-hematopoietic cell types. Since Ubc13 has a broad role in regulating NF-κB signalling, it is crucial to understand how Ubc13 expression is affected in tumour cells as well as tumour-infiltrating and niche-associated populations, and whether STAT3-mediated effects on Ubc13 expression in specific cell types associate with pro- or anti-tumour responses. This information may help maximize therapeutic targeting in cancer. Animals Hematopoietic Stat3 -deficient ( Tg(Tek-cre)12Flv Stat3 f/Δ ) mice were generated by crossing Tg(Tek-cre)12Flv and Stat3 f/f strains [37] . Age- and gender-matched wild-type controls ( Stat3 w/f ) were used as indicated [37] . Il6 −/− ( Il6 tm1Kopf ) mice were obtained from Jackson Labs; Il6 +/+ mice were used as controls. Ube2n f/f mice were kindly provided by Dr Shizuo Akira [38] . Cre-ER Stat3 f/f , Cre-ER Ube2n f/f and Cre-ER Ube2n f/f Stat3 f/f mice were obtained by crossing Rosa26 CreER mice (kindly provided by Dr Yong-Jun Liu) with Stat3 f/f , Ube2n f/f or Ube2n f/f Stat3 f/f animals, respectively. All strains were on the C57BL/6J background; male and female mice aged 5–12 weeks were used. Randomization, blind allocation or exclusion criteria were not utilized. Animals were housed in a specific pathogen-free barrier facility. Experimental procedures were approved by the Institutional Animal Care and Use Committee at UT MD Anderson Cancer Center. Plasmids A 536 bp fragment of the murine Ube2n promoter, encompassing the consensus STATx site, was amplified from mouse genomic DNA and cloned into the pGL3-Basic vector (Promega) to generate the Ube2n reporter (pGL3- Ube2n ). Mutation of the STATx site in the Ube2n reporter was performed with the QuikChange II Site-Directed Mutagenesis Kit (Agilent Technologies) to generate pGL3- Ube2n -mut. Sequences encoding murine STAT3C (a persistently activated isoform, kindly provided by Dr Jim Darnell) or STAT3-TAD (a TAD deletion mutant) were cloned in the pMX-IRES-GFP vector and used as indicated in gene reporter assays. All plasmid inserts were verified by DNA sequencing. Antibodies and cytokines The following antibodies were used at the indicated dilutions for immunoblotting: pJNK (#9251, 1:1,000), p-p38 (#9211, 1:1,000), pERK1/2 (#9101, 1:1,000) and pSTAT3 antibodies (#9131, 1:1,000), obtained from Cell Signaling; JNK (C-17, 1:1,000), p38 (H-147, 1:1,000), ERK1/2 (K-23, 1:1,000), TRAF6 (H-274, 1:1,000), anti-ubiquitin (P4D1, 1:1,000), RAN (C-20, 1:1,000), STAT3 (C-20, 1:1,000), c-Myc (9E10, 1:5,000) and tubulin antibodies (10D8, 1:2,000), obtained from Santa Cruz Biotech; and anti-K63 ubiquitin (HWA4C4, 1:750) and anti-Ubc13 antibodies (#371100, 1:1,000), obtained from Enzo and Invitrogen, respectively. TRAF6 antibody (H-274) was also used for immunoprecipitation (1 μg per sample). For ChIPs, the following antibodies were used at 2 μg per sample: STAT3 (C-20) and c-Ets-1 antibodies (C-20), obtained from Santa Cruz Biotech; H3K4me3 (CS200580) and total H3 antibodies (04-928), obtained from Millipore; and Set1 antibody (A300-289A), from Bethyl Laboratories. For flow cytometry, fluorescently labelled antibodies to CD11b (M1/70, fluorescein isothiocyanate-labelled), F4/80 (BM8, PerCP Cy5.5-labelled), M-CSFR (AFS98, APC-labelled) and RANK (R12-31, phycoerythrin-labelled) from eBioscience were used at a 1:100 dilution. Recombinant murine RANKL, IL-6, IL-10 and IL-6-blocking antibodies were purchased from R&D Systems. Cell lines HEK293T cells and Stat3 −/− MEFs were cultured in Dulbecco’s modified Eagle’s medium (DMEM) containing 10% fetal bovine serum (FBS). L929 cells were cultured in DMEM containing 10% FBS for 7 days to generate macrophage colony-stimulating factor (M-CSF)-containing conditioned medium [39] . HEK293T and L929 were obtained from American Type Culture Collection. Stat3 −/− MEFs were kindly provided by Dr David Levy. Bone marrow cultures and in vitro osteoclastogenesis Bone marrow cells were flushed from femurs and tibia of age-matched mice (5–12 weeks). Bone marrow-derived macrophages were prepared by culturing bone marrow cells in DMEM supplemented with 20% FBS and 30% M-CSF-containing conditioned medium for 4–6 days [39] . In vitro osteoclast differentiation was induced by culturing bone marrow-derived macrophages in M-CSF-conditioned media for 4 days, then adding RANKL (25–100 ng ml −1 ) for additional 3–4 days [40] . Stat3 deletion in vitro To induce Stat3 deletion, 4-hydroxytamoxifen (1 μM, Sigma-Aldrich) was added to macrophage cultures from Cre-ER Stat3 f/f , Cre-ER Ube2n f/f or Cre-ER Stat3 f/f Ube2n f/f mice every 48 h throughout the culture period. As controls, Stat3 f/f macrophages were cultured similarly with 4-hydroxytamoxifen. Flow cytometry Bone marrow-derived macrophages were stained with fluorescently labelled antibodies on ice for 30 min. Cells were analysed by flow cytometry on an LSRII machine (BD Bioscience). Data were further analysed by FlowJo. RNA isolation and qPCR Total RNA was extracted by Trizol and reverse transcribed with iScript (Bio-Rad); qPCR was performed with SYBR Green PCR Mix (Bio-Rad) and a sequence detector (Bio-Rad 5000). The expression of individual genes was calculated and normalized to 18s RNA [37] . Data are presented as fold change between the test groups and controls, as indicated in the figure legends. Gene-specific primers are listed in Supplementary Table I . Immunoprecipitations and immunoblotting For TRAF6 immunoprecipitations, cells were lysed under denaturing conditions and immunoprecipitations were performed with TRAF6-specific antibody in a buffer containing 50 mM Tris, pH 7.4, 150 mM NaCl, 0.1% SDS, 0.5% sodium deoxycholate and 1% Nonidet P-40, supplemented with 1 mM N -ethylmaleimide. Ubiquitinated TRAF6 was detected by immunoblotting with pan-ubiquitin antibodies or antibodies specific for the K63 ubiquitin linkage; total TRAF6 was detected on immunoblots by TRAF6 antibody. For all other immunoblots, whole-cell lysates were generated in RIPA buffer supplemented with a phosphatase inhibitor cocktail (Roche) and subjected to immunoblotting [40] . The relative density of protein signals on immunoblots was measured by NIH Image J software. Full images of immunoblots are shown in Supplementary Figs 7–9 . Electrophoretic mobility shift assays Nuclear extracts were prepared from bone marrow-derived macrophages, and 10 μg of extract was incubated with double-stranded 32 P-radiolabelled probes specific for NF-κB, NF-Y or Oct-1 in 12 μl of electrophoretic mobility shift assay reaction buffer containing 2 μg of poly (dI-dC), 20 mM HEPES (pH 7.9), 1 mM MgCl 2 , 50 mM KCl, 0.05 mM EDTA, 0.5 mM dithiothreitol, 0.05% Igepal-CA630 and 5% glycerol [41] . Protein–DNA complexes were separated on non-denaturing 5% polyacrylamide gels containing 0.5 × Tris-borate-EDTA buffer (45 mM Tris-borate and 1 mM EDTA). Probe sequences are listed in Supplementary Table I . Chromatin immunoprecipitations Bone marrow-derived macrophages were stimulated with IL-6 or IL-10, as indicated in the figure legends. ChIPs were performed with antibodies to STAT3 (Santa Cruz Biotech), H3K4me3 (Millipore), total H3 (Millipore), Set1 (Bethyl Laboratories), c-Ets-1 (Santa Cruz Biotech) or rabbit IgG control (Santa Cruz Biotech) using a ChIP assay kit, as per the manufacturer’s instructions (Millipore). For STAT3, Set1 or c-Ets-1, ChIP results were normalized first to the relevant input sample, and then to the untreated (NT) sample from Stat3 -sufficient cells to determine fold change. For H3K4me3 ChIPs, results were normalized to data from ChIPs with total H3 antibody. Normalized data were plotted versus the corresponding predicted ChIP amplification product from the Ube2n proximal promoter region, as indicated by the schematic diagram in Fig. 5 . Reporter gene assays HEK293T cells were transfected with the Ube2n reporter construct and the indicated plasmids (see Figure legend), using Lipofectamine LTX (Invitrogen) as per the manufacturer’s instructions. Cells were cultured in DMEM for 24–48 h. Luciferase activity was measured with a Dual Luciferase assay kit obtained from Promega using a Sirius luminometer (Berthold Detection Systems) [37] . Statistical analysis Data are presented as mean±s.e.m. The statistical significance between two groups was calculated by a two-tailed t -test. For multiple groups, significance was evaluated by two-way analysis of variance with Bonferroni multiple comparisons. Graphpad Prism 5 software was used for each type of analysis. How to cite this article: Zhang, H. et al. STAT3 restrains RANK- and TLR4-mediated signalling by suppressing expression of the E2 ubiquitin-conjugating enzyme Ubc13. Nat. Commun. 5:5798 doi: 10.1038/ncomms6798 (2014).